Rats track odour trails accurately using a multi-layered strategy with near-optimal sampling Tracking odour trails is a crucial behaviour for many animals, often leading to food, mates or away from danger. It is an excellent example of active sampling, where the animal itself controls how to sense the environment. Here we show that rats can track odour trails accurately with near-optimal sampling. We trained rats to follow odour trails drawn on paper spooled through a treadmill. By recording local field potentials (LFPs) from the olfactory bulb, and sniffing rates, we find that sniffing but not LFPs differ between tracking and non-tracking conditions. Rats can track odours within ∼ 1 cm, and this accuracy is degraded when one nostril is closed. Moreover, they show path prediction on encountering a fork, wide 'casting' sweeps on encountering a gap and detection of reappearance of the trail in 1–2 sniffs. We suggest that rats use a multi-layered strategy, and achieve efficient sampling and high accuracy in this complex task. The ability of animals to track odour trails is well known but sparingly studied [1] , [2] , [3] , [4] , [5] , [6] . Fundamental issues regarding the behavioural and neural mechanisms of this ethologically important behaviour remain poorly understood. These include the possible use of stereo odour sampling, active sampling strategies, and whether neural correlates seen in constrained tasks [7] are present in this more natural behaviour. Rodents are primarily olfactory animals with robust and versatile olfactory learning abilities. However, odour trail tracking in rodents has not been thoroughly studied in the lab. In studies on other animals, a few common themes have emerged. First, as shown clearly by moths, insects often combine zigzagging through an odour plume while approaching its source and wide 'casting' movements to search for the trail whenever they lose it [8] , [9] . The zigzagging approach has been observed in several other animals including bees, cockroaches, dogs and humans [5] , [10] , [11] , [12] . Second, the use of stereo olfaction in efficiently performing this task has been repeatedly suggested. Disrupting bilateral input affects tracking in bees [12] , drosophila larvae [6] , [13] and humans [11] . This behaviour represents a good example of active sensory sampling, where the animal itself modulates when and where it receives sensory input in order to get a better picture of its environment [14] . Here, we describe the development of an experimental system where rats were trained to follow trails of different odours. We show that odour trail tracking employs a multi-layered strategy utilizing near-optimal sampling and path prediction, and develop a model that captures many aspects of this strategy. Further, sniffing and local field potential (LFP) characteristics during this task differ from those seen in more constrained tasks. Rats track various odour trails accurately We trained nine female Wistar rats to track odour trails (see Methods). We built a treadmill that used a 38 cm wide and 3 m long looped sheet of paper as its belt on which the rats ran ( Fig. 1a ). A meandering odour trail was drawn on this paper. The trail was either a pure odourous liquid deposited at a fixed rate on the paper, and was uniformly 3 mm wide ( Supplementary Fig. S1 ), or a chocolate trail where a piece of chocolate was rubbed manually and uniformly on the paper, and was again about 3 mm wide. The liquid odours were L-carveol (LC, spearmint odour) and phenethyl alcohol (PEA, rose odour). These odours were relatively less volatile and were smelled distinctly by the experimenter only when the nose was directly above the trail. Thus by studying 'surface-borne' odour trail tracking, we have circumvented the difficult problem of studying air-borne odour plumes with animals moving through them [1] . 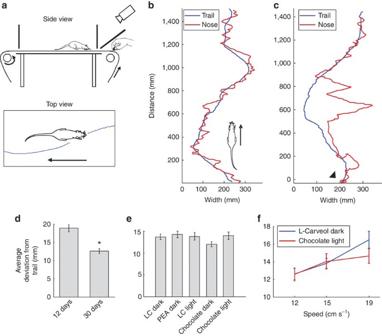Figure 1: Rats can track odour trails on a treadmill. (a) A schematic of the apparatus. Above, a side view of the treadmill showing camera position. Below, top view showing the trail in blue. (b) An example of a stretch of tracking. The rat's nose trajectory (red) is overlaid on the trail (blue) in this and subsequent figures. The rat always moves from the bottom to the top. Note that thexandyscaling in this and subsequent such plots are not always equal. (c) An example where after pausing to eat a chocolate piece (arrowhead), the rat resumed tracking by making wide casting movements to first find the trail. The trails inbandcwere chocolate in light and LC in the dark, respectively. (d) The mean deviation of the nose from the trail compared between 12 and 30 days post initiation of training was significantly reduced, *P< 10−4(two-tailedt-test,P=2.3×10−5,n=21 stretches from four rats andn=19 stretches from four rats, respectively, chocolate trail in light, 12 cm s−1speed). (e) Mean deviations across different trail conditions is constant (analysis of variance,P=0.15, mean deviation=13.8, 14.3, 13.9, 12.0 and 14.0 mm,n=36, 30, 29, 28 and 22 stretches, respectively, and all with four rats except chocolate in light, three rats, all 15 cm s−1speed). (f) Mean deviation at three different treadmill speeds and for two different trails. There was a significant difference only between the 19 cm s−1case and the other two lower speeds for LC in dark trail (analysis of variance followed by a multiple comparison procedure,P=0.0048). Figure 1: Rats can track odour trails on a treadmill. ( a ) A schematic of the apparatus. Above, a side view of the treadmill showing camera position. Below, top view showing the trail in blue. ( b ) An example of a stretch of tracking. The rat's nose trajectory (red) is overlaid on the trail (blue) in this and subsequent figures. The rat always moves from the bottom to the top. Note that the x and y scaling in this and subsequent such plots are not always equal. ( c ) An example where after pausing to eat a chocolate piece (arrowhead), the rat resumed tracking by making wide casting movements to first find the trail. The trails in b and c were chocolate in light and LC in the dark, respectively. ( d ) The mean deviation of the nose from the trail compared between 12 and 30 days post initiation of training was significantly reduced, * P < 10 −4 (two-tailed t -test, P =2.3×10 −5 , n =21 stretches from four rats and n =19 stretches from four rats, respectively, chocolate trail in light, 12 cm s −1 speed). ( e ) Mean deviations across different trail conditions is constant (analysis of variance, P =0.15, mean deviation=13.8, 14.3, 13.9, 12.0 and 14.0 mm, n =36, 30, 29, 28 and 22 stretches, respectively, and all with four rats except chocolate in light, three rats, all 15 cm s −1 speed). ( f ) Mean deviation at three different treadmill speeds and for two different trails. There was a significant difference only between the 19 cm s −1 case and the other two lower speeds for LC in dark trail (analysis of variance followed by a multiple comparison procedure, P =0.0048). Full size image As the treadmill moved, we occasionally placed small pieces of chocolate on the trail. The rats soon learnt to track the odour trail to find the chocolate. All the rats tracked the trail by moving their noses over the trail in a zigzag fashion, similar to the reports for other species [8] , [10] , [11] , [12] ( Fig. 1b, and Supplementary Movie S1 ). They were able to track all the different types of trails closely and were capable of following turns, often correcting their path very rapidly. On losing the trail, rats sometimes made wide sweeping movements ( Fig. 1c ), akin to the casting behaviour observed in moths, when they have lost a scent trail [8] . It also appears that the nose zigzagging movement is not generated by only a neck-onwards movement, but by involving the entire body ( Supplementary Fig. S2 ). In order to characterize the tracking behaviour of rats, we measured the average absolute horizontal distance of the nose from the trail in different stretches of tracking (a 'stretch' and its deviation from the trail are defined in Supplementary Methods ). This mean deviation, or accuracy of tracking, was compared across different conditions. We first checked if rats displayed learning over time. The mean deviation from the trail decreases significantly from 12 days to 30 days after initiating training ( Fig. 1d ). This suggests that this behaviour has a learning component to it. We next studied different types of odour trails. The three substances used for our trails, LC, PEA and chocolate, are clearly distinct odours. In addition, the chocolate trail is different because it leaves a texture of deposited chocolate behind, as opposed to the textureless LC and PEA trails. Further, we also considered the contribution of visual information, by comparing tracking in the light and dark. We thus studied five different trail conditions. Interestingly, all these conditions showed the same level of accuracy ( Fig. 1e ). As the LC and PEA in dark are purely odour trails, this suggests that the other trails are also tracked primarily using odour cues. Further, rats were unable to track an odourless line drawn by pencil in light ( Supplementary Movie S2 ), suggesting that they do not rely on visual cues. Last, we studied different treadmill speeds. There is an increase in the deviation with increasing speeds for both trails studied ( Fig. 1f ). This may be because the trail can veer away from the rat rapidly at higher speeds, and wider nose swings reduce the chance of thus losing the trail. Though deviation consistently increased with speed, there was a significant difference only between the 19 cm s −1 case and the other two lower speeds for the LC in dark trail. Stereo olfaction improves accuracy of tracking Rats have been shown to have stereo olfaction, the ability to localize an odour by comparing the signals across nostrils [15] . Similar abilities have been demonstrated in other animals [2] , [12] , [16] , [17] . It is not known if rats use this ability in the context of tracking odour trails. We tested this by stitching closed one nostril in each of three rats to disrupt bilateral odour sampling. These same rats earlier underwent a sham surgery in which the stitch did not close the nostril. We found that the unilaterally sensing rats were still able to follow odour trails, but they needed to make larger movements over the trail compared with sham controls ( Fig. 2a,b and Supplementary Movie S3 ). The PEA trail was made of approximately double intensity for both sham and stitched cases to compensate for the reduction in the amount of odour reaching the rat when stitched. The deviation from the trail for the stitched rats in both PEA and chocolate trails in dark was significantly higher than sham ( Fig. 2c,d ). Though the complexity of this behaviour makes it difficult to rule out other effects of closing one nostril, we nevertheless suggest that the loss of stereo sampling is a likely factor in this degradation of performance and that stereo sampling may contribute to efficient performance in natural odour tracking. 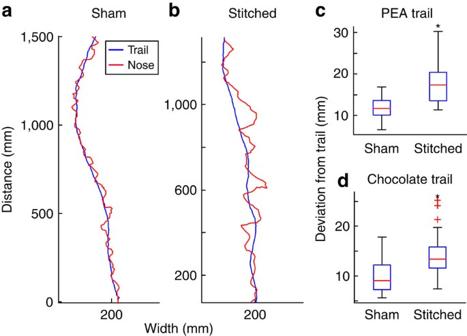Figure 2: Nostril stitching reduces tracking accuracy. (a) An example with a sham stitch. (b) An example of the same rat with the right nostril stitched closed (chocolate trail in dark, 19 cm s−1speed). (c,d) Box plots showing that the median deviation from the trail for the stitched case was significantly higher than sham for both a PEA trail of double intensity (c) and chocolate trail (d), *P< 10−3. Two-tailed Wilcoxon rank-sum test,P=1.56×10−4,n=25 and 17 stretches for PEA sham and stitched, respectively,P=5.95×10−5,n=34 and 27 stretches for chocolate sham and stitched, respectively, 19 cm s−1speed, all with three rats. On box plots here and later, the central mark is the median, the edges of the box are the 25th and 75th percentiles, the whiskers extend to the most extreme data points not considered outliers, and outliers are red crosses. Figure 2: Nostril stitching reduces tracking accuracy. ( a ) An example with a sham stitch. ( b ) An example of the same rat with the right nostril stitched closed (chocolate trail in dark, 19 cm s −1 speed). ( c,d ) Box plots showing that the median deviation from the trail for the stitched case was significantly higher than sham for both a PEA trail of double intensity ( c ) and chocolate trail ( d ), * P < 10 −3 . Two-tailed Wilcoxon rank-sum test, P =1.56×10 −4 , n =25 and 17 stretches for PEA sham and stitched, respectively, P =5.95×10 −5 , n =34 and 27 stretches for chocolate sham and stitched, respectively, 19 cm s −1 speed, all with three rats. On box plots here and later, the central mark is the median, the edges of the box are the 25th and 75th percentiles, the whiskers extend to the most extreme data points not considered outliers, and outliers are red crosses. Full size image Sniffing is modulated during tracking We next utilized the tracking task in conjunction with two physiological measurements. We implanted a thermocouple (TC) in the rat's nasal cavity to monitor the sniffing (five rats), and a LFP electrode in the olfactory bulb (OB) to monitor neural activity (four rats). Example traces of the voltage signals from both are shown in Fig. 3a . An example plot of the sniffing frequency over time shows that the sniffing frequency varied very rapidly from sniff to sniff ( Fig. 3b ). Interestingly, sniffing frequencies were higher and less variable during tracking (black bar in Fig. 3b ). This can also be seen in an example trace with the sniffing frequency overlaid on the nose trajectory in colour code ( Fig. 3c ). 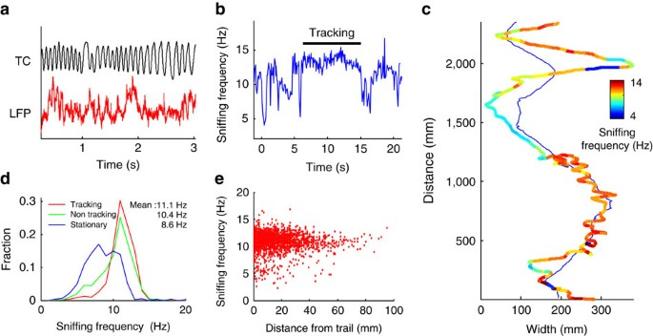Figure 3: Modulation of sniffing during tracking. (a) Example traces of simultaneously recorded sniffing through a thermocouple (TC, black trace) and local field potential signals from the OB (LFP, red trace). (b) Example trace of sniffing frequency over time, calculated at each sniff. Black bar indicates tracking period. (c) An example stretch with the sniffing frequency overlaid on the nose trajectory in colour code. The rat is tracking from about 400 to 1200 mm. Chocolate trail in dark, speed 15 cm s−1. (d) Sniffing frequency histograms of tracking (red) and non-tracking periods (green) at 19 cm s−1(53 stretches each), and with the treadmill stationary (blue, 11 cases). The three distributions are all significantly different (Kruskal Wallis test and multiple comparison procedure,P<10−7). (e) Scatter plot of the sniffing frequency versus the distance from the trail at the time of that sniff. 57 stretches, Pearson's correlation=−0.04. In Fig 3d, we summarize the sniffing frequencies during different behaviours at 19 cm s −1 treadmill speed. This and subsequent data are pooled data from chocolate and PEA trails in dark, unless specified, as they showed no differences. Sniffing frequencies were significantly higher during tracking (11.1±1.7 Hz,), than non-tracking (10.4±2.3 Hz), and were further significantly lower when the treadmill was stationary (8.6±2.4 Hz; during stationary periods, the rat was typically exploring the walls of the box). Sniffing frequency during tracking at a slower 15 cm s −1 speed (10.9±1.9 Hz) was slightly but significantly lower than that at 19 cm s −1 , but still significantly higher than non-tracking periods ( Supplementary Fig. S3 ). In general, the sniffing behaviour observed here is highly dynamic [18] , [19] . Interestingly, the frequencies observed during odour tracking are much higher than the ∼ 8 Hz observed during odour-based discriminations in more-controlled odour sampling tasks in rats [15] , [18] . This higher 11–12-Hz sniffing has been observed in these previous studies but it occurred only during the period of reward anticipation. Figure 3: Modulation of sniffing during tracking. ( a ) Example traces of simultaneously recorded sniffing through a thermocouple (TC, black trace) and local field potential signals from the OB (LFP, red trace). ( b ) Example trace of sniffing frequency over time, calculated at each sniff. Black bar indicates tracking period. ( c ) An example stretch with the sniffing frequency overlaid on the nose trajectory in colour code. The rat is tracking from about 400 to 1200 mm. Chocolate trail in dark, speed 15 cm s −1 . ( d ) Sniffing frequency histograms of tracking (red) and non-tracking periods (green) at 19 cm s −1 (53 stretches each), and with the treadmill stationary (blue, 11 cases). The three distributions are all significantly different (Kruskal Wallis test and multiple comparison procedure, P <10 −7 ). ( e ) Scatter plot of the sniffing frequency versus the distance from the trail at the time of that sniff. 57 stretches, Pearson's correlation=−0.04. Full size image We tested if the sniffing frequency is modulated by how far the rat's nose is from the trail. We found no such correlation ( Fig. 3e ). The correlation coefficient was −0.04 and was not significantly different from 0 (Pearson's correlation, P =0.098). We also plotted sniffing frequency versus nose oscillation phase, or half of one complete zigzag of the nose across the odour trail. This too showed no significant modulation ( Supplementary Fig. S3 ). Further, the sniffing frequency was also not correlated with the nose velocity ( Supplementary Fig. S3 ). LFP oscillations are dynamic and uncorrelated with sniffing We measured the LFP from the OB simultaneously with sniffing in four rats. The raw LFP traces ( Fig. 3a , bottom) showed transient oscillations at a range of frequencies. We studied the frequency bands of theta (4–12 Hz), beta (14–44 Hz) and gamma (60–90 Hz) in further detail. 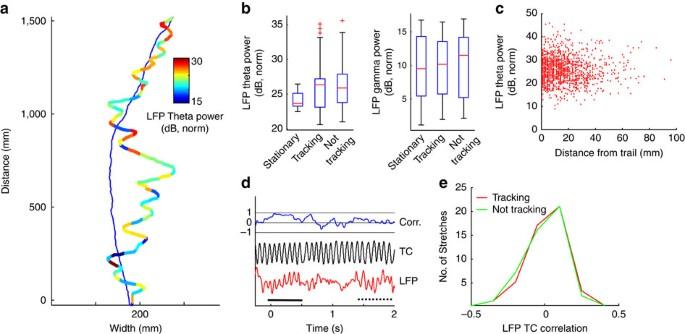Figure 4: Modulation of OB LFP during tracking. (a) An example stretch of tracking with the LFP theta (4–12 Hz) power overlaid on the nose trajectory in colour code. Chocolate trail in dark, 19 cm s−1. (b) Box plots showing that there is no significant difference between tracking and not tracking periods and stationary treadmill periods for theta power (left, Kruskal Wallis test,P=0.10) or gamma power (right, Kruskal Wallis testP=0.97,n=47 stretches in both tracking and not tracking,n=9 for stationary condition). (c) Scatter plot of the LFP theta power (calculated at 128 ms intervals) versus the distance of the nose from the trail. 47 stretches, Pearson's correlation=−0.02. (d) The thermocouple signal (black, TC) and LFP signal (red, LFP) show transient high correlations (blue, Corr.). Both TC and LFP are filtered through a 30 Hz low-pass filter. The correlation is calculated in a 200 ms sliding window. The dotted lines show 0 and ±1 correlation. Solid horizontal line shows a period of theta oscillations with high correlation. Dashed horizontal line shows a period of theta but low correlation. (e) Histograms of correlation coefficients of the TC and LFP signals during tracking (red) and non-tracking (green) periods. The two distributions are not significantly different (47 stretches, two-tailedt-test,P=0.84). Figure 4a shows the power of theta oscillations colour coded on the rat's nose trajectory. Theta oscillations typically varied rapidly over time ( Fig. 4a ). We compared theta power between the stationary treadmill case, the rat tracking case and the case of the rat not tracking but running on the treadmill ( Fig. 4b , left). There was no significant difference between stationary, tracking and not tracking conditions. We also looked at the gamma and beta oscillations across these three conditions and found no significant difference between them ( Fig. 4b , right; Supplementary Fig. S4 ). Figure 4: Modulation of OB LFP during tracking. ( a ) An example stretch of tracking with the LFP theta (4–12 Hz) power overlaid on the nose trajectory in colour code. Chocolate trail in dark, 19 cm s −1 . ( b ) Box plots showing that there is no significant difference between tracking and not tracking periods and stationary treadmill periods for theta power (left, Kruskal Wallis test, P =0.10) or gamma power (right, Kruskal Wallis test P =0.97, n =47 stretches in both tracking and not tracking, n =9 for stationary condition). ( c ) Scatter plot of the LFP theta power (calculated at 128 ms intervals) versus the distance of the nose from the trail. 47 stretches, Pearson's correlation=−0.02. ( d ) The thermocouple signal (black, TC) and LFP signal (red, LFP) show transient high correlations (blue, Corr.). Both TC and LFP are filtered through a 30 Hz low-pass filter. The correlation is calculated in a 200 ms sliding window. The dotted lines show 0 and ±1 correlation. Solid horizontal line shows a period of theta oscillations with high correlation. Dashed horizontal line shows a period of theta but low correlation. ( e ) Histograms of correlation coefficients of the TC and LFP signals during tracking (red) and non-tracking (green) periods. The two distributions are not significantly different (47 stretches, two-tailed t -test, P =0.84). Full size image We tested if the LFP oscillations were modulated by how far the nose was from the trail. Such modulation would be expected if there was a significant odour-driven oscillation when the nose was directly above the trail. To test this, we plotted the LFP theta power versus the distance from the trail ( Fig. 4c ). The correlation was −0.02 and was not significantly different from 0 (Pearson's correlation, P =0.13). This result was the same for the gamma and beta oscillations as well ( Supplementary Fig. S4 ). Together, these data suggest that the LFP oscillations in the OB are not strongly modulated by the tracking behaviour or the olfactory input during this task. The OB LFP oscillations have been considered to be highly correlated with the animal's respiration or sniffing [20] , [21] , [22] . However, it has been shown in the rat whisker system that though the whisking frequency and hippocampal theta oscillations have the same frequencies, they are not synchronous [23] . We similarly determined the extent of correlation between the TC and LFP signals. We first calculated the correlation between the raw TC and LFP electrode signals in a 200-ms sliding window. The sniffing and LFP signals showed transient periods of high correlations (example trace in Fig. 4d , solid horizontal line shows the period of high correlation). However, we could not find any consistent behavioural correlate of these short high-correlation stretches. Further, there were other periods with LFP oscillations of similar frequency as sniffing, which showed no correlation with it (dashed horizontal line). We then calculated the average correlation between the two signals for each stretch of tracking. We did the same for equivalent stretches where the rat was not tracking. The histograms of the values of these correlations are shown in Fig. 4e (47 stretches each). The values were low, with the mean for tracking periods being 0.007 and for non-tracking periods being 0.004. Further, the two distributions were not significantly different. Overall, we find no correlations between sniffing and LFP under any of our behavioural contexts. Rats scan gaps widely and predict bifurcation trail direction In order to better understand the strategies rats use to follow these trails, we presented them with two variations of the simple trail-tracking task. In the first case there was a gap in the trail. All the six rats tested in this condition showed a strong tendency to increase the width of their nose swings on encountering the gap. 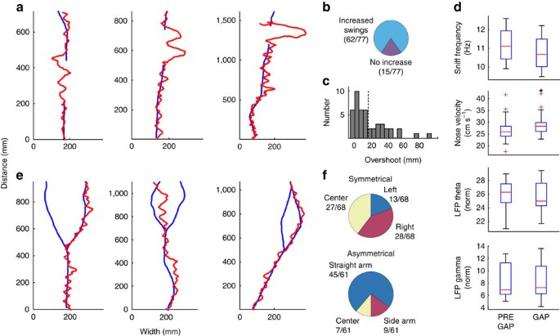Figure 5: Trails with gaps and bifurcations. (a) Examples of encountering a gap in the trail. The rats increased the amplitude of their nose swings. The gap was 23 cm wide on a chocolate trail in dark and speed was 15 cm s−1in all three. (b) Pie chart showing that in 62/77 or 80.5% of the cases there was at least a doubling in the swing amplitudes on encountering the gap. (c) Histogram of the distance of overshoot on the first pass on the trail on resuming tracking after the gap. Dotted line indicates the 15 mm limit, which included 61% of the cases. (d) Box plots comparing the gap period and an equal duration period just preceding the gap. Plots show the sniffing frequency (19 stretches, four rats), nose velocity (47 stretches, five rats), LFP theta oscillations (14 stretches, three rats) and LFP gamma oscillations (14 stretches, three rats). Only the nose velocity was significantly increased during the gap period (two-tailed Wilcoxon rank-sum test,P=0.002 for nose velocity,P>0.05 for the rest, all with 19 cm s−1speed). (e) Examples of encountering a bifurcation in the trail. The rat could choose one of the arms of the bifurcation (left, chocolate trail in dark, 15 cm s−1) or neither and go though the centre (centre, chocolate trail, 19 cm s−1). If one of the arms of the bifurcation was going in roughly the same direction as the approaching stretch ('Straight Arm'), the rats preferred that arm (right, chocolate trail, 19 cm s−1). (f) Pie charts show the distribution of behaviours observed for symmetrical bifurcations (above) and asymmetrical bifurcations (below). Figure 5a shows three examples of this behaviour (see also Supplementary Movie S4 ). In 62/77 or 80.5% of the cases, there was at least a doubling of the width of the nose swing on encountering the gap ( Fig. 5b ). As soon as they re-encountered the trail, they resumed tracking with very little overshoot. Of all cases where tracking was resumed, 61% overshot by <15 mm ( Fig. 5c ), which is comparable to the average distance from the trail during normal tracking. Further, in 67% of cases it took <120 ms to reverse the movement of the nose on re-encountering the trail. Given that these rats sniff at ∼ 11 Hz, this suggests that they make this decision in one to two sniffs. Thus, wide casting behaviour is a reliable fallback strategy on losing the trail, and the rat can very rapidly return to on-trail tracking when it finds the trail. Figure 5: Trails with gaps and bifurcations. ( a ) Examples of encountering a gap in the trail. The rats increased the amplitude of their nose swings. The gap was 23 cm wide on a chocolate trail in dark and speed was 15 cm s −1 in all three. ( b ) Pie chart showing that in 62/77 or 80.5% of the cases there was at least a doubling in the swing amplitudes on encountering the gap. ( c ) Histogram of the distance of overshoot on the first pass on the trail on resuming tracking after the gap. Dotted line indicates the 15 mm limit, which included 61% of the cases. ( d ) Box plots comparing the gap period and an equal duration period just preceding the gap. Plots show the sniffing frequency (19 stretches, four rats), nose velocity (47 stretches, five rats), LFP theta oscillations (14 stretches, three rats) and LFP gamma oscillations (14 stretches, three rats). Only the nose velocity was significantly increased during the gap period (two-tailed Wilcoxon rank-sum test, P =0.002 for nose velocity, P >0.05 for the rest, all with 19 cm s −1 speed). ( e ) Examples of encountering a bifurcation in the trail. The rat could choose one of the arms of the bifurcation (left, chocolate trail in dark, 15 cm s −1 ) or neither and go though the centre (centre, chocolate trail, 19 cm s −1 ). If one of the arms of the bifurcation was going in roughly the same direction as the approaching stretch ('Straight Arm'), the rats preferred that arm (right, chocolate trail, 19 cm s −1 ). ( f ) Pie charts show the distribution of behaviours observed for symmetrical bifurcations (above) and asymmetrical bifurcations (below). Full size image We also recorded sniffing and LFP while the rats performed the gap task. We calculated the average sniffing frequency, nose velocity, and theta and gamma power in the LFP signal before and during the gap ( Fig. 5d ). Of these, the nose velocity showed a significant increase during the gap due to the casting behaviour, while the remaining measures showed no difference. In another variation, we presented six rats with a bifurcation in the trail ( Fig. 5e , Supplementary Movie S5 ). This bifurcation was either symmetrical ( Fig. 5e left, centre) or asymmetrical, where one of the two arms continued in approximately the same direction, that is, the straight arm ( Fig. 5e , right). In each case, the rats either chose one of the two arms or went through the centre. The distributions among these behaviours are shown in Fig. 5f . Interestingly, upon encountering an asymmetrical bifurcation, the rats had a strong preference to proceed along the arm that was going straighter ( Fig. 5f ). This, and the tendency to continue straight through the centre in symmetrical bifurcations ( Fig. 5f ), suggests that in our setup the trail-tracking strategy has a predictive component, where the rat expects the trail to continue in the same direction. Rats use a highly efficient gradient measurement strategy We next asked how a rat might combine nose position and the sniffing times in its sampling strategy. We first checked if the combination of rate of sniffing and nose oscillations was optimized by some mathematical criterion. To do this, we plotted each sniff overlaid on the trajectory of the nose ( Fig. 6a ), designating the time from the valley to the peak of the TC signal as inhalation and peak to next valley as exhalation. This plot shows that the rat typically sniffs multiple times in each cyclic sweep, or nose oscillation, across the odour trail. We took a subset of stretches, which had relatively consistent nose oscillations, and measured the number of sniffs per nose oscillation. The histogram of these values is shown in Fig. 6b . The average is 5.7 sniffs per nose oscillation, or 2.85 sniffs each time the nose crosses the trail. This is close to the optimal Shannon–Nyquist sampling criterion of two samples per cycle (the Shannon–Nyquist theorem is a result from information theory that states that the rate of sampling a signal need be only twice its highest frequency in order to completely determine the signal). This number is constant for two different treadmill velocities tested ( Supplementary Methods ). Though it is unlikely that the rat is estimating an odour concentration time series in the rigorous sense of information theory, this result is none the less indicative of a highly efficient strategy. In fact, close to two sniffs per trail crossing suggests a comparison across only a pair of samples before making a decision to turn. 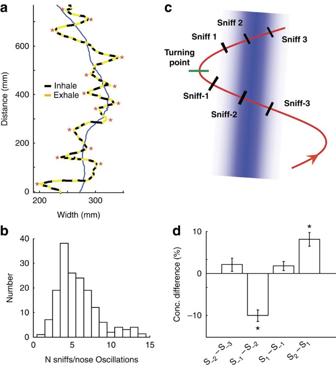Figure 6: Sampling strategies. (a) An example stretch of tracking showing each sniff overlaid on the nose trajectory. Black indicates inhalation and yellow exhalation. Multiple sniffs are taken during each nose oscillation. (b) Histogram of the number of sniffs per nose oscillation (33 stretches combining 15 and 19 cm s−1cases). (c) A schematic of the nose crossing the trail showing the location of a turning point and the locations at which sniffs were taken. (d) Values of the difference in concentration detected on average between two consecutive sniffs (percentage of the maximum concentration, 34 stretches,t-test, *P<0.05). S−1refers to the Sniff-1 in panelcand so on. Figure 6: Sampling strategies. ( a ) An example stretch of tracking showing each sniff overlaid on the nose trajectory. Black indicates inhalation and yellow exhalation. Multiple sniffs are taken during each nose oscillation. ( b ) Histogram of the number of sniffs per nose oscillation (33 stretches combining 15 and 19 cm s −1 cases). ( c ) A schematic of the nose crossing the trail showing the location of a turning point and the locations at which sniffs were taken. ( d ) Values of the difference in concentration detected on average between two consecutive sniffs (percentage of the maximum concentration, 34 stretches, t -test, * P <0.05). S −1 refers to the Sniff-1 in panel c and so on. Full size image This highly efficient tracking behaviour prompted us to look at the sampling strategy in further detail. We asked how many sniffs it takes going down a falling odour gradient before the rat decides to reverse direction. Here, we considered the nose turning point and the sniffs before and after it ( Fig. 6c ). As we know the location of the nose at the time of each sniff, we can estimate the concentration of odour at each sniff if we know the concentration cross-section of the trail. As the rat's nostrils have added 'reach' on each side due to the air flow patterns [24] , we chose the effective trail cross-section to be a Gaussian of s.d. 20 mm. The following results, however, are also valid for narrower and broader trails (7 mm to 50 mm). We calculated the average difference in odour concentration detected by the rat in the two sniffs just before it turned (S −1 –S −2 ) and the two sniffs just before these (S −2 –S −3 ). These values are plotted in the first two bars in Fig. 6d . The average difference detected just before a turn (S −1 –S −2 ) was significantly different from zero (−9.9% of the maximum concentration). Interestingly, the difference between the two sniffs just preceding this (S −2 –S −3 ) is not significantly different from zero (2.1%). Thus, on an average, the rat uses only a pair of sniffs to detect a drop in the concentration that prompts it to reverse its direction. The remaining two bars in Fig. 6d show the differences in concentration detected by later sniffs. The sniffs just before and after a turn do not detect a significant difference (mean difference 1.8%). The sniff pair just after this, however, does encounter a significant difference (mean difference 8.1%). Thus, on average, the rat uses just two sniffs to detect a rise in concentration when it moves towards the trail. Judging from the above results, it appears that rats indeed have a near-optimal sampling strategy. Rats do not favour 'off centre' edge tracking For an animal tracking an odour trail, the rising and falling odour concentration at the edges of the trail contains more information than the centre of the trail. Using this logic, a recent study has predicted that the zigzagging of a rat's nose should be centred on the edge of the trail and not on its centre, similar to bats directing their ultrasonic clicks on the edges of objects instead of directly at them [25] . We tested this prediction by measuring the mean of the rat's nose trajectory with respect to the trail. With the narrow trails studied so far, we found many stretches where the nose was not centred on the trail, but consistently to one side ( Fig. 7a ). We plotted the mean of the nose and its error for four rats that tracked a trail of LC in the dark ( Fig. 7b ). Interestingly, all four rats showed a significantly rightward-shifted tracking trajectory ( t -test, P <0.05). Data from other trails showed similar trends, including the nostril stitched case. 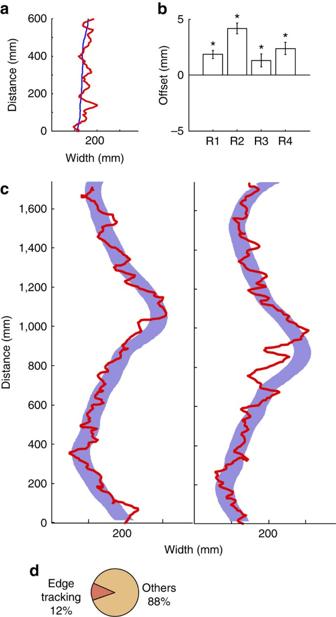Figure 7: Off-centre tracking and wide trails. (a) An example stretch of tracking of a chocolate trail (∼3 mm wide) showing the nose trajectory centred to the right of the trail, yet consistently crossing the trail. (b) The average offsets from 3 mm wide trails across 67 stretches for four rats (R1–R4) tracking an LC trail in the dark, all three speeds combined. Positive values indicate a bias to the right of the trail. All rats showed a significant rightward shift of the nose from the trail (t-test, *P<0.05, error bars represent s.e.m.). Similar effects were observed for all trails studied. (c) Two example stretches of rats tracking an extra-wide chocolate trail (45 mm wide). (d) Only 12% of the total tracking duration was classified as edge tracking. The rest of the time the rat appeared to utilize multiple different strategies (22 stretches, four rats, 19 cm s−1speed). Figure 7: Off-centre tracking and wide trails. ( a ) An example stretch of tracking of a chocolate trail ( ∼ 3 mm wide) showing the nose trajectory centred to the right of the trail, yet consistently crossing the trail. ( b ) The average offsets from 3 mm wide trails across 67 stretches for four rats (R1–R4) tracking an LC trail in the dark, all three speeds combined. Positive values indicate a bias to the right of the trail. All rats showed a significant rightward shift of the nose from the trail ( t -test, * P <0.05, error bars represent s.e.m.). Similar effects were observed for all trails studied. ( c ) Two example stretches of rats tracking an extra-wide chocolate trail (45 mm wide). ( d ) Only 12% of the total tracking duration was classified as edge tracking. The rest of the time the rat appeared to utilize multiple different strategies (22 stretches, four rats, 19 cm s −1 speed). Full size image However, this is not proof of edge tracking, as the nose still crosses over to the other side of the trail consistently ( Fig. 7a ). To test for edge tracking, we used a much wider trail (a 45 mm wide chocolate trail, with a step-shaped odour profile, Supplementary Movie S6 ). Two examples of nose trajectories are shown in Fig. 7c . These show a complex strategy that involved not only zigzagging on the trail edge but also zigzagging completely across the entire trail, and to a greater extent, moving inside the trail till hitting the edge and then turning. In fact, the percentage of edge tracking (locking onto and zigzagging across one edge) was only 12% ( Fig. 7d ). Thus, although detecting the edges of a trail is critical to tracking, rats do not appear to do purely edge tracking. Quantitative model of path prediction and error estimates We developed a mathematical and computer model to test and refine our understanding of the rat odour tracking strategy. This model involved the rat's nose moving at a constant forward velocity and a constant x-velocity across the trail until deciding to turn. The model rat obtained noisy, discrete samples of the odour concentration and its gradient, akin to sniffing, at 11 Hz. It also maintained an estimate of where the trail was and an error in that estimate. It would turn around if one of the following happened: (a) it detected a large drop in odour concentration (comparing with previous sniff), (b) it detected a large downward gradient of odour (in that sniff) or c) it crossed beyond the trail error estimate. Details of the model are in the Supplementary Methods . We implemented this model in Matlab. The resulting computer simulations qualitatively resembled observed tracking behaviour well ( Fig. 8a,b ). Specifically, it replicated the tracking of meandering trails ( Fig. 8a ), an increase in the deviation from the trail when stereo sampling was lost ( Fig. 8a inset), the casting behaviour upon encountering a gap ( Fig. 8b ) and choosing one arm in a bifurcation ( Fig. 8c left), with a preference for the straight branch in asymmetrical bifurcations ( Fig. 8c right, inset. Tracking continues down the straight arm in 70% of cases.). 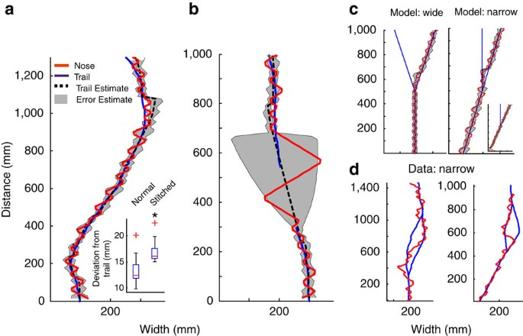Figure 8: Model of tracking. (a) An example trace of a simulated nose trajectory tracking a meandering trail. The black dashed line is the rat's estimate of the position of the trail and the grey region indicates its estimate of the error in the trail position, that is, the limits of where it thinks the trail can be. The trail estimate can veer away from the true trail at turns, as in the real tracking cases. Inset: box plots showing that on removing odour gradient information from the model, similar to stitching one nostril closed, the simulated deviation from the trail increases (median deviation from trail increases significantly from 12.5 mm to 16.2 mm, 24 stretches each, two-tailed Wilcoxon rank-sum test,P=8.04×10−6). (b) An example of the model's behaviour on encountering a gap in the trail. The error estimate starts to grow and the nose makes wider swings until it crosses the error estimates. On re-encountering the trail, the error estimate is reset and the tracking resumes. (c) Left: on encountering a wide bifurcation, the model continues tracking down one of the arms, with equal probability of choosing left or right in symmetrical bifurcations. Right: for narrow bifurcations, the model switches between the two arms in 25% of cases. Inset: In 70% of cases for asymmetrical bifurcations, tracking proceeds along the straight arm. (d) Experimental data showing switching on narrow bifurcations, which happens in 27% of cases. PEA and chocolate trail in dark, respectively, speed 19 cm s−1. Figure 8: Model of tracking. ( a ) An example trace of a simulated nose trajectory tracking a meandering trail. The black dashed line is the rat's estimate of the position of the trail and the grey region indicates its estimate of the error in the trail position, that is, the limits of where it thinks the trail can be. The trail estimate can veer away from the true trail at turns, as in the real tracking cases. Inset: box plots showing that on removing odour gradient information from the model, similar to stitching one nostril closed, the simulated deviation from the trail increases (median deviation from trail increases significantly from 12.5 mm to 16.2 mm, 24 stretches each, two-tailed Wilcoxon rank-sum test, P =8.04×10 −6 ). ( b ) An example of the model's behaviour on encountering a gap in the trail. The error estimate starts to grow and the nose makes wider swings until it crosses the error estimates. On re-encountering the trail, the error estimate is reset and the tracking resumes. ( c ) Left: on encountering a wide bifurcation, the model continues tracking down one of the arms, with equal probability of choosing left or right in symmetrical bifurcations. Right: for narrow bifurcations, the model switches between the two arms in 25% of cases. Inset: In 70% of cases for asymmetrical bifurcations, tracking proceeds along the straight arm. ( d ) Experimental data showing switching on narrow bifurcations, which happens in 27% of cases. PEA and chocolate trail in dark, respectively, speed 19 cm s −1 . Full size image The model also made an interesting prediction. On encountering a wide bifurcation, it chose one of the two arms and stuck to it ( Fig. 8c left), but for narrow bifurcations (such as the asymmetrical bifurcations), in 25% of cases it went down one arm and then switched to the other ( Fig. 8c right). We looked for this pattern in the experimental data and found that indeed in 27% of the narrow bifurcation cases there was switching between the two arms (for example, Fig. 8d , Supplementary Movie S5 ). This was not seen in any wide bifurcations (for example, Fig. 5e left), thus validating the above prediction. Our study is among the first to combine behavioural and physiological measurements in an animal tracking an odour trail. We find that rats can rapidly track surface-borne odours with highly efficient, near-optimal sampling, and achieve this high performance using a combination of strategies. Stereo sampling improves tracking precision significantly, and rats employ complementary search strategies such as path prediction and casting to follow trails and recover from errors. We are able to model these strategies and find that path prediction accounts for many details of the observed tracking behaviour. Sniffing rates during tracking are among the highest reported for any olfactory task and are modulated continually and rapidly. Our study provides significant insights into the neuroethology of odour trail tracking. We believe that this behaviour of odour trail tracking on a treadmill is close to a natural and ethologically relevant one. The key 'natural' aspect of behaviour in our task is that the rat controls when and where sensory sampling occurs, and guides its movements accordingly. In addition, this complex behaviour emerged spontaneously, without explicit training. We only placed chocolate pieces on the trail, and the rats quite rapidly discovered that the best strategy was to track the trail to find the chocolate. This basic pattern of movement is seen in moths, dogs and humans tracking unrestrained in the open [8] , [10] , [11] , [26] . Furthermore, we were able to characterize the underlying strategies used by the rats. The rats had the fallback of casting behaviour on losing the trail, an assumption of the trail continuing in a straight direction, a sampling rate that matched their movement pattern to provide efficiency and a stereo nostril comparison to further improve accuracy. Also, they did not track only the edge of a wide trail as had been predicted [25] . Thus it is a repertoire of behaviours connected with rules (in short, a strategy) that the rats bring to this task. This supports the claim that we are studying a naturally relevant behaviour. The salient differences between the current task and natural behaviour are the fact that the rat is on a treadmill instead of a true track, that the speed at which the rat may move forward is governed by the treadmill speed and the finite width of the treadmill box. Further, the speed of the treadmill was much slower than the maximum speed at which a rat runs, which is about 1 m s −1 (unpublished results). The ability of animals to compare across two nostrils or antennae has been shown in various species, including rats, flies, humans and moths [12] , [15] , [16] , [17] . However, it was not known if animals use this ability to track odours. Our study provides evidence for a direct link between stereo olfaction and natural olfactory behaviours. The sniffing data provide useful insights into sampling strategies during tracking. First, the sniffing frequency is on an average at 10–12 Hz, the highest sniffing frequency reported across rats and mice [18] , [19] . This finding clears doubts about the use of this high-frequency sniffing in a relevant context [27] . Second, rats could detect the resumption of the trail after a gap, within just 1–2 sniffs. Third, the sniffing rate combined with the nose movement is optimized for efficiently tracking the trail. Thus, a sniff is not only a snapshot of the olfactory world [27] but a stereo snapshot whose location and timing are dynamically modulated for highly efficient sampling. The LFP oscillations provided us neural correlates of this complex behaviour. Running on the treadmill elicited a small but insignificant increase in the theta power compared with the stationary condition. Previous studies in many animals including rats [7] , [28] , hedgehogs [29] , zebrafish [30] , locusts [31] and mollusks [32] have found an increase in LFP oscillations at various frequency ranges on odour stimulation. Given this background, it is surprising that we found no difference between the conditions of tracking and not tracking for any frequency band. Even when comparing across conditions when the nose was close to or far from the trail, we saw no difference. Another significant finding of the present study was that the LFP theta oscillation is not strongly correlated with sniffing. This correlation has been shown in anaesthetized rats but is prominent only during odour presentation [20] . In awake animals there was some previously reported evidence for correlations [21] . This lack of increased oscillations or correlations with sniffing is interesting, and though largely unexplained at present, may be related to the fact that the rats are constantly running/walking in our experiments. In the present study, we suggest that active sampling is guided by an internal model of the world. By computationally modelling this internal representation, we suggest that, in addition to position and direction of the odour trail, there is likely to be a representation of uncertainty of position. We suggest that the orbitofrontal cortex, in combination with the hippocampus, may be a likely candidate for neuronal activity encoding representations of the odour trail. The hippocampus has been shown to have olfactory [33] , [34] as well as spatial representations [35] . The orbitofrontal cortex has been shown to encode uncertainty [36] . These parameters may be revealed by further studies involving single-unit recordings from these brain regions. Animals All of the experimental procedures were approved by the National Centre for Biological Sciences institutional animal ethics committee, in accordance with the guidelines of the Government of India and equivalent guidelines of the Society for Neuroscience. Nine female Wistar rats were used for this experiment. The rats were 3 months old at the start of the training. Males could not be used because they soon grew too heavy for the treadmill to pull. Apparatus and odour trails The treadmill was constructed using parts from an old dot matrix printer. The basic design is shown in Fig. 1a . A stepper motor located at the rear end of the treadmill turned a rod that pulled a sheet of dot matrix paper perforated at the sides. The paper passed through a transparent Perspex box, which had gaps in the bottom of the front and back walls to allow the paper to pass through. The box was 380 mm wide and 500 mm long. The paper was also 380 mm wide. The paper was looped around in most experiments. The length of the loop was usually 3 m and occasionally slightly more. As the treadmill was running with the rat on it, the experimenter placed pieces of chocolate on the paper before it entered the box through the gap and became available to the rat. A cardboard was placed to obscure the rat's view of the chocolate being placed. A camera was used to film this from a top-front angle at 25 frames per second. The camera could film in visible light as well as infrared light in which case the arena was lit with an array of infrared light-emitting diodes. The odours LC and PEA were chosen for the odour trails because they were appropriately volatile ( Supplementary Methods ). Also, PEA is known not to excite the trigeminal nerve, which is sensitive to irritant chemicals, even at high concentrations. Thus, this task utilizes only the main olfactory pathway. These trails were made by depositing the chemical at a constant rate on the paper in a meandering line. Chocolate trails were also used and were drawn by rubbing a chocolate piece over the paper. Surgical procedures For nostril stitching and sham stitching, rats were placed under surgical plane halothane anaesthesia (Surgivet) for 10 min after which the nose cone providing anaesthetic was removed from the rat. This provided about 1 min before the rat started to recover during which the stitch was made. For the nostril stitch, one stitch was made using cotton suture closing the nostril completely. The closure of the nostril was checked by placing a drop of water on the closed nostril. For the sham stitch, a stitch was made that did not close the nose but just looped through the upper flap of the nostril. First, the sham stitch was done on the left nostril of three rats that were tested 5.5 h later the same day. A week later, the same rats underwent nostril stitching on the right nostril and were again tested 5.5 h later. Stitches were removed the same evening or next morning. For implanting the TC and LFP electrode, surgery was performed under halothane anaesthesia maintained at a surgical plane and regularly monitored by a lack of response to a sharp toe pinch. Halothane was used at 4% for induction and adjusted between 1.25–2% for maintenance. Rectal temperature was measured and maintained by a heating lamp at about 95° F. Five rats were implanted with both TCs and LFP electrodes; one of them gave no LFP signals. The two wires from the TC, the LFP electrode (and reference if present) and ground wire were connected to a light-weight connector, which was cemented on the rat's skull using 6–8 skull screws. Post surgery, the site was cleaned with iodine solution, neomycin sulphate antibiotic powder was applied and 5 mg kg −1 pentazocine (an analgesic) was injected subcutaneously. The pentazocine was given every 12 h for about 2 days. The rat was allowed to recover for at least 5 days before resuming the behavioural tasks. Electrophysiology During recording sessions, the TC and LFP signals were first passed through a custom-made head-mounted preamp and then through a tether, and were amplified further in a commercial amplifier (Neuralynx Inc.). The TC signal was differentially amplified from ×10,000 to ×200,000 depending on the signal quality. The LFP was amplified with respect to a skull screw in three rats and with respect to a reference electrode in the OB in one rat. LFP signals were generally amplified from ×2,000 to ×5,000 depending on the signal quality. The LFP signal was filtered in the amplifier from 1–200 Hz. The signals were digitized at 1,000 Hz and stored on a computer (DAP 5200a data acquisition card, Microstar Laboratories). Video analysis The video of the rat tracking was taken from the front and at an elevated angle at 25 frames per second (Sony Handycam DCR-SR300E, Sony Corporation). We first chose sections of the video through visual inspection where the rat was tracking the trail. The criterion for choosing a section of video was that the rat should be following the trail with its nose on the paper for at least 2 s. As the rat usually moved its nose zigzag when it was on the paper, the criterion was effectively that its nose should be crisscrossing the trail consistently for at least 2 s. Usually short stretches just before and after the tracking were included here. The time spent not tracking was spent in zigzagging its nose on non-trail areas, pausing to eat chocolate crumbs and rearing up against or sniffing the side and front walls, as seen in Supplementary Movie S2 . We took a video from a side angle and confirmed that the rats were not licking the chocolate trail while they were tracking. The video selections, typically 4–10 s, were then digitized using custom software in Matlab (MathWorks Inc.). We took each frame, and found the position of the trail and the rat's nose. To do this, we first performed a projective transformation of the region described by the four corners of the box. This prevented errors in calculating coordinates owing to the rat being at different distances from the camera. The trail was detected automatically at the front edge, and the user had to click on the tip of the rat's nose for each frame. The error in the manual estimation of the nose by this method was calculated by doing this for the same stretch of ∼ 50 frames ten times. The error (s.d.) was 1 mm in both x and y coordinates. How to cite this article: Khan, A.G. et al . Rats track odour trails accurately using a multi-layered strategy with near-optimal sampling. Nat. Commun. 3:703 doi: 10.1038/ncomms1712 (2012).